Proteolysis of MOB1 by the ubiquitin ligase praja2 attenuates Hippo signalling and supports glioblastoma growth Human glioblastoma is the most frequent and aggressive form of brain tumour in the adult population. Proteolytic turnover of tumour suppressors by the ubiquitin–proteasome system is a mechanism that tumour cells can adopt to sustain their growth and invasiveness. However, the identity of ubiquitin–proteasome targets and regulators in glioblastoma are still unknown. Here we report that the RING ligase praja2 ubiquitylates and degrades Mob, a core component of NDR/LATS kinase and a positive regulator of the tumour-suppressor Hippo cascade. Degradation of Mob through the ubiquitin–proteasome system attenuates the Hippo cascade and sustains glioblastoma growth in vivo . Accordingly, accumulation of praja2 during the transition from low- to high-grade glioma is associated with significant downregulation of the Hippo pathway. These findings identify praja2 as a novel upstream regulator of the Hippo cascade, linking the ubiquitin proteasome system to deregulated glioblastoma growth. Gliomas are malignant brain tumours that arise from glial cells. They are the most common primary proliferative disorders of the central nervous system in the adult population. They include a heterogenous group of tumours that are characterized by a variety of differentiation and malignant phenotypes [1] . Glioblastoma multiform (GBM), which represents about 50% of total gliomas, is the most aggressive form of brain tumour, with a very poor median survival after initial diagnosis [2] . High-grade gliomas are thought to derive from low-grade variants. These variants undergo sequential genetic alterations, giving rise to cell populations with more invasive behaviour, greater activation of mitogenic pathways and loss of cell cycle control [3] . Transition from low- to high-grade glioma is also marked by activation of the hypoxia pathway, which promotes blood vessel formation, clonal evolution and consequent tumour expansion [4] , [5] , [6] , [7] , [8] , [9] , [10] . At the molecular level, GBMs are characterized by a wide array of genetic and epigenetic alterations. The pathogenic role of these abnormalities in glioma development has been functionally confirmed by in vivo studies. Thus, inactivation of tumour suppressor genes (p53), constitutive activation of membrane receptors (EGFR), induction of prosurvival pathways (PI3K/Akt), aberrant gene transcription and metabolic dysfunction have all been linked mechanistically to the development and progression of GBMs [3] , [11] , [12] , [13] , [14] , [15] , [16] , [17] . These abnormalities underlie the high recurrence rate and resistance of these tumours to current therapies. Although major advances have been made recently in identifying the relevant players that regulate GBM growth and development, so far the key mechanisms and the genes responsible of glial neoplastic transformation remain subjects of active investigation. The ubiquitin–proteasome system (UPS) is emerging as an important control mechanism of cell metabolism, growth and survival. The UPS is the principal pathway for eliminating unneeded or damaged proteins [18] . UPS couples ubiquitylation of a target protein to its proteolytic cleavage. Ubiquitylation is a multistep process that involves the sequential action of three enzymes: activating enzymes (E1), conjugating enzymes (UBCs or E2s) and ligases (E3s). E3-ubiquitin ligases fall into two main classes characterized by a HECT domain or a RING domain [19] , [20] . HECT domain E3 ligases act catalytically to form a thioester intermediate during ubiquitin transfer to substrate, whereas RING E3 ligases serve as a scaffold that brings together the substrate and the E2 ligase. praja2 belongs to a growing family of mammalian RING E3-ubiquitin ligases widely expressed in cells and several tissues, including brain [21] , [22] . praja2 finely tunes the stability of intracellular substrates and has a significant role in critical aspects of cell signalling [23] . During cAMP stimulation, praja2 promotes ubiquitin-dependent proteolysis of the inhibitory protein kinase A (PKA) regulatory (Rs) subunits, sustaining downstream PKA signalling and significantly impacting on gene transcription and neuronal activity [24] . However, the role of praja2 in tumour cell growth and the relevant molecular targets involved are unknown. Here, we report a mechanism of signal attenuation in human GBM based on proteolytic turnover of components of the tumour-suppressor Hippo pathway. We find that praja2 directly binds to and ubiquitylates Mps one binder 1 (MOB1), a component and core effector of the Hippo pathway. Degradation of ubiquitylated MOB1 by the proteasome inhibits this signalling cascade, favoring GBM growth. By manipulating the levels and activity of praja2, we have uncovered a pivotal role of this ligase in glial cell tumorigenesis. praja2 interacts with Hippo pathway component MOB1 To gain insight into praja2 function, we performed a yeast two-hybrid screening using a human brain cDNA library and the C-terminal domain of praja2 as bait. Two independent clones encoding the C-terminus of MOB1 co-activator protein were isolated. MOB1 is a core component of the nuclear-Dbf2-related kinase 1 (NDR1)/LATS (large tumour suppressor) kinase complex that acts as a downstream effector of the Hippo pathway. Hippo is an evolutionally conserved protein kinase cascade that has a fundamental role in the control of cell growth and organ size [25] . First, we set out to verify the direct interaction of MOB1 and praja2 detected in the two-hybrid screen. We confirmed that praja2 directly binds to MOB1 in vitro . A fusion protein carrying full-length praja2 fused to the C-terminus of glutathione S -transferase polypeptide (GST) coprecipitated in vitro -translated [ 35 S]-labelled MOB1 ( Supplementary Fig. S1a ). Reciprocal experiments using purified, recombinant GST-MOB1 confirmed interaction with praja2 expressed in HEK293 cells ( Supplementary Fig. S1b ). Co-immunoprecipitation assays showed that exogenous flag-praja2 and co-expressed HA-MOB1 formed a stable complex ( Fig. 1a ). As praja2 promotes degradation of MOB1 (see below), we treated the cells for 12 h with the proteasome inhibitor MG132 before harvesting in order to see the complex. Deletion mutagenesis and binding assays identified residues 531–630 as the praja2 segment that interacts with MOB1 ( Fig. 1a ). Next, we demonstrated this interaction in vivo by isolating endogenous praja2/MOB1 complex from cell lysates. LATS1 kinase was also present in the praja2 precipitates ( Fig. 1b ). In vitro binding assays showed that MOB1A is required for praja2–LATS1 interaction ( Fig. 1c ). The MOB1-binding domain relies within a region of praja2 that is also involved in PKA R interaction. Therefore, we tested if PKA binding to praja2 was affected by MOB1. The results indicate that this is, indeed, the case. Thus, PKA–praja2 interaction was significantly reduced by coexpression of exogenous MOB1A ( Supplementary Fig. S2a,b ). As consequence, PKA inactive holoenzyme accumulates in cells expressing MOB1A ( Supplementary Fig. S2c,d ). 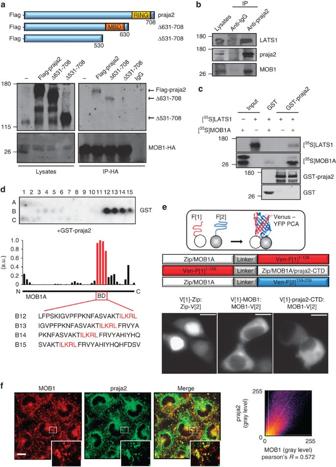Figure 1: praja2 forms a complex with MOB1. (a) Schematic representation of the praja2 constructs used (upper panel). HEK293 cells were transiently transfected with HA-MOB1A and flag-tagged praja2 (either wild-type or deletion mutants). Cells were treated for 12 h with MG132 (10 μM) before harvesting. Twenty-four following transfection, cells were harvested and lysed. Lysates were subjected to immunoprecipitation with anti-HA antibody. Precipitates were immunoblotted with anti-HA and flag antibodies (lower panels). (b) Endogenous praja2/MOB1/LATS1 complex was isolated from cell lysates using anti-praja2 antibody. (c)In vitro-translated [35S]-labelled MOB1A and LATS1 were subjected to pulldown assays with purified GST or GST–praja2 fusion. (d) Spotted peptides (25 mers, 20 aa overlap) of MOB1A were overlaid with recombinant GST-praja2 followed by immunoblotting with anti-GST. The bar graph illustrates the densitometric quantification of the average ofn=2 dot blot experiments, coloured bars indicate the sequences (red box, referred here as binding domain (BD)) of one potential binding site in the illustrated modular structure of MOB1A. (e) Schematic view of the principle of the Venus-YFP PCA to capture protein complexes directly in the living cell and of the fusion proteins (indicated as circles) tested. Fluorometric imaging of transiently transfected HEK293 cells co-expressing the indicated proteins tagged with Venus-YFP PCA fragment (1) or (2) 24 h post transfection (lower panels). Scale bar, 10 μm. (f) U87MG cells were subjected to double immunostaining with monoclonal anti-MOB1 and polyclonal anti-praja2 antibodies. Images were collected and analysed by confocal microscopy. Magnification of selected areas is shown (insets). Scale bar, 10 μM. Figure 1: praja2 forms a complex with MOB1. ( a ) Schematic representation of the praja2 constructs used (upper panel). HEK293 cells were transiently transfected with HA-MOB1A and flag-tagged praja2 (either wild-type or deletion mutants). Cells were treated for 12 h with MG132 (10 μM) before harvesting. Twenty-four following transfection, cells were harvested and lysed. Lysates were subjected to immunoprecipitation with anti-HA antibody. Precipitates were immunoblotted with anti-HA and flag antibodies (lower panels). ( b ) Endogenous praja2/MOB1/LATS1 complex was isolated from cell lysates using anti-praja2 antibody. ( c ) In vitro -translated [ 35 S]-labelled MOB1A and LATS1 were subjected to pulldown assays with purified GST or GST–praja2 fusion. ( d ) Spotted peptides (25 mers, 20 aa overlap) of MOB1A were overlaid with recombinant GST-praja2 followed by immunoblotting with anti-GST. The bar graph illustrates the densitometric quantification of the average of n =2 dot blot experiments, coloured bars indicate the sequences (red box, referred here as binding domain (BD)) of one potential binding site in the illustrated modular structure of MOB1A. ( e ) Schematic view of the principle of the Venus-YFP PCA to capture protein complexes directly in the living cell and of the fusion proteins (indicated as circles) tested. Fluorometric imaging of transiently transfected HEK293 cells co-expressing the indicated proteins tagged with Venus-YFP PCA fragment (1) or (2) 24 h post transfection (lower panels). Scale bar, 10 μm. ( f ) U87MG cells were subjected to double immunostaining with monoclonal anti-MOB1 and polyclonal anti-praja2 antibodies. Images were collected and analysed by confocal microscopy. Magnification of selected areas is shown (insets). Scale bar, 10 μM. Full size image To map the binary interaction sites, we performed a peptide spotting experiment, first to confirm interaction in vitro and second to determine specific amino acids required for praja2 binding to MOB1A. Overlapping 25-mer peptides derived from human MOB1 were spotted onto a membrane and overlaid with purified GST-praja2 531–631 fusion proteins as previously described [26] . We identified one potential binding site located at the C-terminus of MOB1A with the binding motif ILKRL as the core region for binding ( Fig. 1d ). To test if the C-terminal region of praja2 (amino acids 531–708) interacts with MOB1A in a cellular context, we applied a protein-fragment complementation assay (PCA) based on the ‘Venus’ mutant of the yellow fluorescent protein (YFP) [27] . This assay is independent of a continuous stimulus; the irreversibility of this Venus-YFP PCA will trap transient protein complexes directly in the living cell [26] . Binding of the two proteins brings the unfolded fragments of the YFP-based reporter protein into proximity, allowing for folding and reconstitution of the fluorescent reporter to localize binary protein complexes in vivo [27] ( Fig. 1e , upper panel). As shown in Fig. 1e (lower panels), we were able to detect MOB1A:praja2-CTD (praja2 C-terminal domain, residues 531–708) complexes in vivo . In contrast to the mainly nuclear localisation of the positive control for the protein:protein interaction of a leucine zipper dimer (Zip:Zip), the MOB1A homodimer was cytoplasmic [28] . Accordingly, we detected cytoplasmic complexes between MOB1A-VenF[2] and praja2-CTD N-terminal tagged with YFP PCA VenF[1] ( Fig. 1e ). In situ immunostaining analysis of U87MG glioblastoma cells revealed partial colocalization of endogenous praja2 and MOB1. Overlapping signals were detected at the perinuclear region and in the cytoplasm ( Fig. 1f ), and also at centrosomal region as shown by triple labelling with anti-MOB1, anti-praja2 and anti- γ tubulin antibody ( Supplementary Fig. S3a ). A similar immunostaining pattern was also observed in FNP8, a primary culture of human GBM ( Supplementary Fig. S3b ). praja2 ubiquitylates and degrades MOB1 We postulated that praja2 ubiquitylation promotes MOB1 degradation. We tested this hypothesis by measuring MOB1 levels in cells co-transfected with expression vectors encoding for flag-praja2 (either wild-type or RING mutant) and HA-tagged MOB1. We used two highly conserved variants of MOB1, MOB1A and MOB1B. As shown in Fig. 2a , expression of wild-type praja2 significantly reduced HA-MOB1A levels relative to the CMV vector control. In contrast, transfection with the inactive praja2 mutant (praja2rm) increased the concentration of HA-MOB1A. Similar results were obtained with co-transfected MOB1B ( Fig. 2c ). Endogenous MOB1 was also efficiently degraded by transfected praja2 ( Fig. 2e ). Treatment with MG132 reversed the reduction by praja2 of the levels of HA-MOB1A ( Fig. 2f ) or of endogenous MOB1 ( Fig. 2g ). To demonstrate that praja2 affected MOB1 stability, rather than MOB1 synthesis, the experiments were repeated in presence of cycloheximide, an inhibitor of protein synthesis. 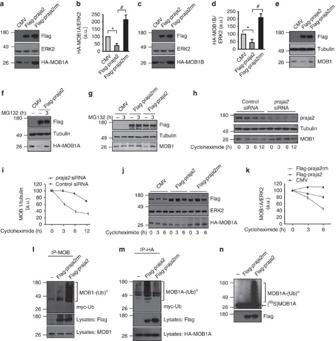Figure 2: praja2 ubiquitylates and degrades MOB1. (a–d) HEK293 cells were transiently co-transfected with CMV or flag-praja2 (either wild-type or RING mutant) and HA-MOB1A (a) or HA-MOB1B (c) vectors. Lysates were immunoblotted with the indicated antibodies. Quantitative analysis (mean±s.e.m) is reported in the panels (b,d), respectively. *P<0.01 versus CMV;#P<0.01 versus flag-praja2, Student’st-test. (e) Immunoblot analysis of endogenous MOB1 on lysates from cells transiently transfected with CMV, flag-praja2 or flag-praja2rm vector. Tubulin was used as loading control. (f) Cells were transiently co-transfected with CMV or flag-praja2 and HA-MOB1A vectors. Lysates were immunoblotted with the indicated antibodies. The cells were treated for 8 h with MG132 (20 μM) before harvesting. (g) Cells were transiently transfected with CMV or flag-praja2 (either wild-type or RING mutant) and treated for 8 h with MG132 (20 μM) before harvesting. Lysates were immunoblotted with the indicated antibodies. (h) Cells transiently transfected with control siRNA orpraja2siRNA were treated with cycloheximide and harvested at the indicated time points after treatment. Lysates were immunoblotted with the indicated antibodies. (i) Cumulative analysis (mean±s.e.m.) of the experiments shown inh. (j) Cells transiently co-transfected with HA-MOB1A and with either the expression vector for praja2 or praja2rm. CMV vector was included as control. Lysates were immunoblotted with the indicated antibodies. (k) Cumulative analysis of the experiments shown inj. The data are expressed as mean±s.e.m. of three independent experiments. (l) Cells were transiently co-transfected with myc-ubiquitin and flag-praja2 or flag-praja2rm. Cells were treated for 8 h with MG132 (20 μM) before harvesting. Lysates were immunoprecipitated with anti-MOB1 antibody. The precipitates and lysates were immunoblotted with anti-MOB1, anti-myc and anti-flag antibodies. (m) Same as inl, except cells were transiently co-transfected with HA-MOB1A and lysates were immunoprecipitated with anti-HA antibody. Precipitates and lysates were immunoblotted with anti-HA, anti-myc and anti-flag antibodies. (n)In vitro-translated, [35S]-labelled MOB1A was incubated with flag-praja2 or flag-praja2rm (immunopurified from transfected cells) and his6-tagged ubiquitin, in the presence of E1 and UbcH5c (E2). The reaction mixture was denatured, size-fractionated on 12% SDS–PAGE, and analysed by autoradiography. A fraction of the reaction mixture was immunoblotted with anti-flag antibody (lower panel). Figure 2h shows that MOB1 levels declined over time in control cells, with a half-life of ~5 h. Knocking down endogenous praja2 significantly increased the half-life of endogenous MOB1 ( Fig. 2h ) and of HA-MOB1A ( Supplementary Fig. S4a,b ). Complementary experiments demonstrated that praja2 overexpression markedly reduced HA-MOB1A stability ( Fig. 2j ), whereas endogenous MOB1 ( Supplementary Fig. S4c,d ) or HA-MOB1 ( Fig. 2j ) were stabilized by praja2rm overexpression. Figure 2: praja2 ubiquitylates and degrades MOB1. ( a – d ) HEK293 cells were transiently co-transfected with CMV or flag-praja2 (either wild-type or RING mutant) and HA-MOB1A ( a ) or HA-MOB1B ( c ) vectors. Lysates were immunoblotted with the indicated antibodies. Quantitative analysis (mean±s.e.m) is reported in the panels ( b , d ), respectively. * P <0.01 versus CMV; # P <0.01 versus flag-praja2, Student’s t -test. ( e ) Immunoblot analysis of endogenous MOB1 on lysates from cells transiently transfected with CMV, flag-praja2 or flag-praja2rm vector. Tubulin was used as loading control. ( f ) Cells were transiently co-transfected with CMV or flag-praja2 and HA-MOB1A vectors. Lysates were immunoblotted with the indicated antibodies. The cells were treated for 8 h with MG132 (20 μM) before harvesting. ( g ) Cells were transiently transfected with CMV or flag-praja2 (either wild-type or RING mutant) and treated for 8 h with MG132 (20 μM) before harvesting. Lysates were immunoblotted with the indicated antibodies. ( h ) Cells transiently transfected with control siRNA or praja2 siRNA were treated with cycloheximide and harvested at the indicated time points after treatment. Lysates were immunoblotted with the indicated antibodies. ( i ) Cumulative analysis (mean±s.e.m.) of the experiments shown in h . ( j ) Cells transiently co-transfected with HA-MOB1A and with either the expression vector for praja2 or praja2rm. CMV vector was included as control. Lysates were immunoblotted with the indicated antibodies. ( k ) Cumulative analysis of the experiments shown in j . The data are expressed as mean±s.e.m. of three independent experiments. ( l ) Cells were transiently co-transfected with myc-ubiquitin and flag-praja2 or flag-praja2rm. Cells were treated for 8 h with MG132 (20 μM) before harvesting. Lysates were immunoprecipitated with anti-MOB1 antibody. The precipitates and lysates were immunoblotted with anti-MOB1, anti-myc and anti-flag antibodies. ( m ) Same as in l , except cells were transiently co-transfected with HA-MOB1A and lysates were immunoprecipitated with anti-HA antibody. Precipitates and lysates were immunoblotted with anti-HA, anti-myc and anti-flag antibodies. ( n ) In vitro -translated, [ 35 S]-labelled MOB1A was incubated with flag-praja2 or flag-praja2rm (immunopurified from transfected cells) and his6-tagged ubiquitin, in the presence of E1 and UbcH5c (E2). The reaction mixture was denatured, size-fractionated on 12% SDS–PAGE, and analysed by autoradiography. A fraction of the reaction mixture was immunoblotted with anti-flag antibody (lower panel). Full size image Since praja2 is an E3-ubiquitin ligase, we asked if praja2 ubiquitylates MOB1 in living cells. Indeed, flag-praja2 promoted accumulation of poly-ubiquitylated forms of endogenous MOB1 ( Fig. 2l ) and of the co-transfected HA-MOB1A ( Fig. 2m ). Ligase activity was required for HA-MOB1A ubiquitylation; expression of praja2rm did not enhance MOB1 modification ( Fig. 2l ). An in vitro ubiquitylation assay confirmed that MOB1 is, in fact, a direct substrate of praja2 ( Fig. 2n ). praja2 negatively regulates the Hippo pathway YAP nuclear factor drives transcription of several genes. These include cyclin E and cyclin D, which induce quiescent cells to enter the cell cycle [29] , [30] , [31] . Upon reaching cell confluence and/or defined organ size, activated Hippo/MST phosphorylate the MOB1/LATS dimer, which leads to the activation of MOB1/LATS ( [32] ). Active MOB1/LATS complex phosphorylates YAP transcription factor at S127 ( [32] ). Phosphorylated YAP is trapped within the cytoplasm via interaction with 14-3-3 proteins and eventually degraded. Cytoplasmic sequestration of phosphorylated YAP suppresses the proliferating and antiapoptotic program, leading to cell cycle arrest and inhibition of organ or tumour growth [33] , [34] . We postulated that praja2, by reducing MOB1 levels, would downregulate LATS activity, decreasing YAP phosphorylation and negatively impacting on the downstream Hippo cascade. We tested this idea by monitoring YAP phosphorylation at S127 (pYAP) and MOB1 levels in growing and in quiescent U87MG glioblastoma cells. As control cells reached confluence, YAP phosphorylation increased ~1.7-fold over baseline levels ( Fig. 3a ). Downregulation of endogenous praja2 ( praja2 small interfering RNA (siRNA)) increased the levels of MOB1 and concomitantly enhanced YAP phosphorylation above control siRNA values ( Fig. 3a ). This was associated with marked reduction of YAP accumulation in the nuclei of praja2 siRNA-transfected cells ( Fig. 3c ). Direct interference with endogenous praja2 activity reproduced the effects of praja2 silencing. Thus, expression of the praja2rm mutant increased the levels of MOB1 and enhanced confluence-induced YAP phosphorylation ( Fig. 3e ). As a read-out of YAP transcriptional activity, we measured the levels of cyclin E mRNA [35] , [36] , [37] . As expected, silencing of praja2 significant reduced cyclin E expression, both in U87MG cells and in primary cultures of human GBM (FNP8) ( Fig. 3f ). 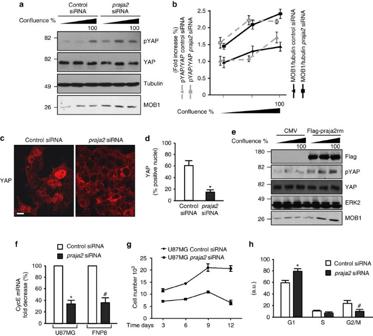Figure 3: praja2 inhibits the Hippo pathway and is required for GBM cell growth. (a) HEK293 cells were transiently transfected with the indicated siRNAs and harvested at different confluence. Lysates were immunoblotted with the indicated antibodies. (b) Cumulative analysis of the experiments shown ina. (c) cells were transiently transfected with siRNAs and subjected to immunostaining with monoclonal anti-YAP. Images were collected and analysed by confocal microscopy. Scale bar, 20 μm. (d) Quantitative analysis (mean±s.e.m) of the experiments shown in (c), *P<0.01 versus control siRNA, Student’st-test. (e) As ina, except the cells were transfected with flag-praja2rm or control CMV plasmid. (f) U87MG and FNP8 cells were transiently transfected with siRNAs and harvested at the indicated time points. Total RNA was extracted and subjected to RT–qPCR analysis for cyclin E (cycE) mRNA expression. Quantitative analysis is shown. These data are expressed as mean±s.e.m. of three independent experiments. *P<0.01 versus control siRNA (U87MG);#P<0.02 versus control siRNA (FNP8), Student’st-test. (g) Growth curve of U87MG siRNA-transfected cells. Following transfection, cells were seeded in multiwell plates, harvested at the indicated time points and counted. A mean value ±s.e.m. of three experiments is shown. (h) Fluorescent-activated cell sorter analysis (FACS) of U87MG cells prepared as inc. The analysis was performed at 48 h following transfection. *P<0.05 versus control siRNA (G1);#P<0.05 versus control siRNA (G2/M). Figure 3: praja2 inhibits the Hippo pathway and is required for GBM cell growth. ( a ) HEK293 cells were transiently transfected with the indicated siRNAs and harvested at different confluence. Lysates were immunoblotted with the indicated antibodies. ( b ) Cumulative analysis of the experiments shown in a . ( c ) cells were transiently transfected with siRNAs and subjected to immunostaining with monoclonal anti-YAP. Images were collected and analysed by confocal microscopy. Scale bar, 20 μm. ( d ) Quantitative analysis (mean±s.e.m) of the experiments shown in ( c ), * P <0.01 versus control siRNA, Student’s t -test. ( e ) As in a , except the cells were transfected with flag-praja2rm or control CMV plasmid. ( f ) U87MG and FNP8 cells were transiently transfected with siRNAs and harvested at the indicated time points. Total RNA was extracted and subjected to RT–qPCR analysis for cyclin E (cycE) mRNA expression. Quantitative analysis is shown. These data are expressed as mean±s.e.m. of three independent experiments. * P <0.01 versus control siRNA (U87MG); # P <0.02 versus control siRNA (FNP8), Student’s t -test. ( g ) Growth curve of U87MG siRNA-transfected cells. Following transfection, cells were seeded in multiwell plates, harvested at the indicated time points and counted. A mean value ±s.e.m. of three experiments is shown. ( h ) Fluorescent-activated cell sorter analysis (FACS) of U87MG cells prepared as in c . The analysis was performed at 48 h following transfection. * P <0.05 versus control siRNA (G1); # P <0.05 versus control siRNA (G2/M). Full size image praja2 is required for cell proliferation and tumour growth in vivo The finding that praja2 downregulates the Hippo pathway provided a starting point to analyse how praja2 contributes to the phenotype of GBM cells. Hippo pathway activity is negatively correlated with growth and aggressive phenotype of GBM [38] . We predicted, therefore, that praja2 inactivation of MOB1 would enhance glial cell transformation. First, we compared praja2 expression in FNP8 and in U87MG cells. Supplementary Figure S5a shows that praja2 is expressed at comparable levels in both cell types. To link causally praja2 to glioma cell malignancy, we asked how praja2 silencing affected cell growth. siRNA duplexes targeting human praja2 efficiently knocked-down endogenous protein ( Supplementary Fig. S5a ). Importantly, downregulation of praja2 markedly inhibited growth of both U87MG ( Fig. 3g ) and FNP8 ( Supplementary Fig. S5b ) cells. The requirement of praja2 for cell growth was confirmed by fluorescent-activated cell sorter analysis. Thus, praja2 siRNA-transfected U87MG cells accumulated at the G1 phase of cell cycle ( Fig. 3h ). A reduction at G2-M transition was also evident in the praja2-silenced cells. Taken together, these findings indicate that praja2 supports the growth of cultured GBM cells. We further tested this notion in vivo using a mouse model of cancer growth. In this model, U87MG cells are injected subcutaneously into CD1 nude mice. The cells start to grow at the site of injection several days post-implantation [39] . To prove that praja2 is, in fact, required for tumour growth in vivo , we silenced endogenous praja2 in U87MG cells before injection by transient transfection with siRNA duplexes targeting praja2 ( praja2 siRNA) or with control non-targeting siRNAs (control siRNA). Three weeks post-injection, the mice were killed and the weight of the lesions was scored. As shown in Fig. 4a , downregulation of praja2 significantly inhibited tumour growth. Similar results were obtained using primary cultures of human GBM (NMDP7) ( Supplementary Fig. S6 ). We also probed the tumour sections for Ki67, a proliferative marker and predictive parameter of glioblastoma recurrence and progression. The number of Ki67-positive cells was reduced by two-fold in tumour sections derived from praja2 siRNA-transfected relative to cells transfected with control siRNA ( Fig. 4a ). The levels of the cyclin-dependent kinase inhibitor p21, a molecular marker of G1 growth arrest, were significantly higher in praja2 siRNA-treated tumours, compared with controls ( Fig. 4c ), confirming the requirement of praja2 for cell cycle progression. 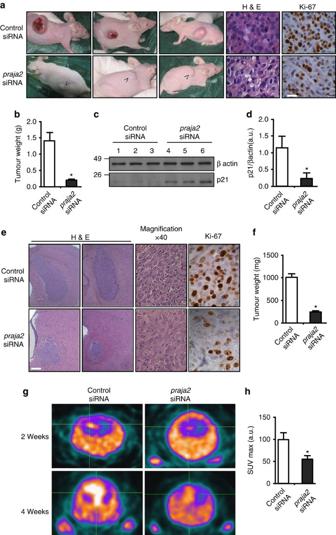Figure 4: praja2 is required for tumour growthin vivo. (a) U87MG cells transiently transfected with siRNAs were subcutaneously implanted into CD1 nude mice. Four weeks later, the mice were killed and the tumours excised and weighed. Tumour sections were fixed and doubly stained with hematoxylin/eosin or subjected to immunohistochemistry with anti-Ki67 antibody. Scale bar, 20 μm. (b) Cumulative data of tumour weight are expressed as mean±s.e.m. Twenty mice for each experimental group were used. *P<0.01 versus control siRNA, Student’st-test. (c) Lysates from tumour lesions described inawere immunoblotted with anti-p21 (cyclin-dependent kinase (CDK) inhibitor) and anti-β actin antibodies. (d) Quantitative analysis of p21 levels in tumour lysates are expressed as mean±s.e.m. of three independent experiments. *P<0.01 versus control siRNA, Student’st-test. (e) U87MG cells transiently transfected with control siRNA orpraja2siRNA were stereotaxically implanted into the brain (left caudate nucleus) of nude mice. Tissue sections from tumour lesions were stained with hematoxylin/eosin or immunostained with anti-Ki67. Scale bar, 400 μm. (f) Quantitative analysis of the experiments shown ine. Data are expressed a mean value±s.e.m. (Control siRNA:n=15,praja2siRNA:n=10). *P<0.01 versus control siRNA, Student’st-test. (g) FLT-PET analysis was performed at 2 and 4 weeks post-implantation. (h) Quantitative analysis of the experiment (at 2 weeks) shown ing. Data are expressed as mean value +/- s.e.m. *P<0.05 versus control siRNA, Student’st-test. Figure 4: praja2 is required for tumour growth in vivo . ( a ) U87MG cells transiently transfected with siRNAs were subcutaneously implanted into CD1 nude mice. Four weeks later, the mice were killed and the tumours excised and weighed. Tumour sections were fixed and doubly stained with hematoxylin/eosin or subjected to immunohistochemistry with anti-Ki67 antibody. Scale bar, 20 μm. ( b ) Cumulative data of tumour weight are expressed as mean±s.e.m. Twenty mice for each experimental group were used. * P <0.01 versus control siRNA, Student’s t -test. ( c ) Lysates from tumour lesions described in a were immunoblotted with anti-p21 (cyclin-dependent kinase (CDK) inhibitor) and anti-β actin antibodies. ( d ) Quantitative analysis of p21 levels in tumour lysates are expressed as mean±s.e.m. of three independent experiments. * P <0.01 versus control siRNA, Student’s t -test. ( e ) U87MG cells transiently transfected with control siRNA or praja2 siRNA were stereotaxically implanted into the brain (left caudate nucleus) of nude mice. Tissue sections from tumour lesions were stained with hematoxylin/eosin or immunostained with anti-Ki67. Scale bar, 400 μm. ( f ) Quantitative analysis of the experiments shown in e . Data are expressed a mean value±s.e.m. (Control siRNA: n =15, praja2 siRNA: n =10). * P <0.01 versus control siRNA, Student’s t -test. ( g ) FLT-PET analysis was performed at 2 and 4 weeks post-implantation. ( h ) Quantitative analysis of the experiment (at 2 weeks) shown in g . Data are expressed as mean value +/- s.e.m. * P <0.05 versus control siRNA, Student’s t -test. Full size image To study the role of praja2 in tumour development in a more physiological tissue context, we used an orthotopic glioblastoma model. U87MG cells transiently transfected with siRNAs ( praja2 siRNA or control siRNA) were implanted stereotaxically into the left caudate nucleus of mouse brain. The mice were killed 3 weeks later. Histological analysis of post-mortem control mouse brain revealed an homogenous tumour mass with sharp borders that was clearly delimited from the adjacent normal brain tissue. The orthotopic tumour, like the subcutaneous tumour, was composed mostly of large pleomorphic cells with abundant eosinophilic cytoplasm ( Fig. 4e ). Exposure of tumour cells to praja2 siRNA, dramatically reduced tumour weight ( Fig. 4e ). A two-fold reduction of Ki67 immunoreactive signal in these tumours further supports the role of praja2 in regulating GBM cellular proliferation ( Fig. 4e ). Growth of GBM lesions in living mice was monitored by positron emission tomography (PET) using the radiolabeled thymidine analogue 18F-fluorothymidine ( 18 F-FLT). 18 F-FLT-PET analysis is routinely used in vivo to trace cell proliferation in a milieu of intact tumour tissue [40] . FLT-PET scanning analysis revealed a two-fold reduction of 18 F-FLT uptake by tumours derived from praja2 siRNA-transfected cells compared with controls ( Fig. 4g ). These findings provide further evidence that praja2 enhances glioma growth in vivo . The praja2-MOB1 axis controls glioma growth in vivo The data presented above indicate that accumulation of praja2 is positively correlated with glioma growth in vitro and in vivo . As MOB1 is a praja2 substrate, we hypothesized that degradation of MOB1 by praja2 inhibits the Hippo pathway, thus enhancing GBM growth. This hypothesis is supported by several additional findings. First, knock-down of praja2 significantly upregulated MOB1 in transplanted U87MG tumours ( Fig. 5a and b ). Second, concomitant downregulation of MOB1 restored growth of praja2-silenced glioblastoma cells ( Fig. 5c ). Downregulation of praja2 activated the Hippo pathway, as shown by increased autophosphorylation of LATS1 at its activation site serine 909 (pLATS1) ( Fig. 5d ) and phosphorylation of YAP at S127 ( Fig. 5d ). This parallels a global downregulation of cyclins. The replication cyclins, cyclin E and cyclin D were downregulated 10-fold and 4.8-fold, respectively, in praja2-silenced cells. Some downregulation of cyclin B (3.6-fold) was also observed ( Fig. 5d ). Consistent with our hypothesis, concomitant downregulation of MOB1 partially reversed the increase in LATS1 and YAP1 phosphorylation induced by praja2 silencing ( Fig. 5d ) Simultaneous knock-down of MOB1 partially restored cyclin expression in the praja2 knock-down cells, particularly in the case of cyclin E, whose expression increased 5.9-fold. These data along with those reported in Fig. 3 suggest that praja2 primarily regulates G1-S progression. Lastly, inhibition of the Hippo signalling by MOB1 knock-down restored tumour growth of praja2-silenced glioblastoma cells in mouse brain ( Fig. 5f ). 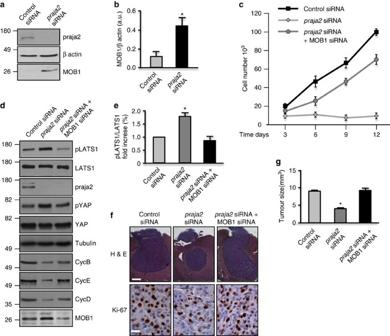Figure 5: The praja2-MOB1 pathway controls tumour growth. (a) Immunoblot analysis for MOB1 on lysates of tumour lesions excised from mice inoculated with siRNA-transfected U87MG cells. (b) Quantitative analysis of the experiments shown ina. Data are expressed as a mean value ±s.e.m. *P<0.01 versus control siRNA, Student’st-test. (c) Growth curve of U87MG siRNA-transfected cells. Following transfection, cells were seeded in multiwell plates, harvested at the indicated time points and counted. A mean value ±s.e.m. is shown. (d) U87MG cells were transfected with the indicated siRNAs. Lysates were immunoblotted with the indicated antibodies. (e) Quantitative analysis of autophosphorylation of LATS1 shown ind. *P<0.01 versus control siRNA, Student’st-test. (f) U87MG cells transiently transfected with control siRNA,praja2siRNA orpraja2siRNA, andMOB1siRNA were stereotaxically implanted into the brain (left caudate nucleus) of CD1 nude mice. Tissue sections from tumour lesions were stained with hematoxylin/eosin. Scale bar, 400 μm (upper) and scale bar, 20 μm (lower). (g) Cumulative analysis of the experiments shown inf. Number of animals tested: control siRNA:n=5;praja2siRNA:n=5;praja2siRNA+MOB1siRNA:n=6. *P<0.01 versus control siRNA andpraja2siRNA/MOB1siRNA, Student’st-test. Figure 5: The praja2-MOB1 pathway controls tumour growth. ( a ) Immunoblot analysis for MOB1 on lysates of tumour lesions excised from mice inoculated with siRNA-transfected U87MG cells. ( b ) Quantitative analysis of the experiments shown in a . Data are expressed as a mean value ±s.e.m. * P <0.01 versus control siRNA, Student’s t -test. ( c ) Growth curve of U87MG siRNA-transfected cells. Following transfection, cells were seeded in multiwell plates, harvested at the indicated time points and counted. A mean value ±s.e.m. is shown. ( d ) U87MG cells were transfected with the indicated siRNAs. Lysates were immunoblotted with the indicated antibodies. ( e ) Quantitative analysis of autophosphorylation of LATS1 shown in d . * P <0.01 versus control siRNA, Student’s t -test. ( f ) U87MG cells transiently transfected with control siRNA, praja2 siRNA or praja2 siRNA, and MOB1 siRNA were stereotaxically implanted into the brain (left caudate nucleus) of CD1 nude mice. Tissue sections from tumour lesions were stained with hematoxylin/eosin. Scale bar, 400 μm (upper) and scale bar, 20 μm (lower). ( g ) Cumulative analysis of the experiments shown in f . Number of animals tested: control siRNA: n =5; praja2 siRNA: n =5; praja2 siRNA+ MOB1 siRNA: n =6. * P <0.01 versus control siRNA and praja2 siRNA/ MOB1 siRNA, Student’s t -test. Full size image praja2 is overexpressed in human glioma Given its positive role in glioma cell proliferation and xenograft tumour growth, we investigated the expression profile of praja2 in human gliomas. Tissue samples obtained from first biopsies of patients that underwent brain surgery for low-grade astrocytoma or GBM were homogenized and the protein lysates were immunoblotted with anti-praja2 antibody. Low levels of praja2 were detected in lysates from human astrocytomas, whereas praja2 concentrations were two-fold to three-fold higher in lysates from GBM samples ( Fig. 6a ). Quantitative RT–PCR analysis demonstrated that praja2 mRNA was increased in tumour biopsies of GBM, compared with astrocytoma II ( Fig. 6c ). This was not a consequence of amplification of the praja2 gene in GBM lesions, as shown by fluorescence in situ hybridization ( Supplementary Fig. S7a,b ). Next, we performed immunohistochemistry on tissue sections derived from GBM and astrocytoma patients. The results were consistent with the immunoblotting data. Thus, more praja2 accumulated in GBM compared with astrocytoma tissues ( Fig. 6d ). MOB1 staining inversely correlated with glioma malignancy and praja2 levels. In particular, low-grade astrocytoma cells displayed a strong MOB1 signal that was diffusely distributed throughout the cytoplasm, whereas significantly lower concentrations of MOB1 were detected in GBM cells ( Fig. 6d ). 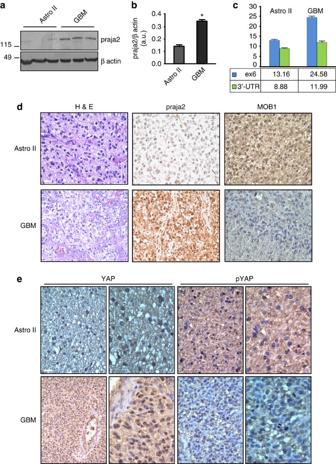Figure 6: praja2 is overexpressed in high-grade human glioma. (a) Lysates from tissue samples of astrocytoma (grade II) and GBM were immunoblotted with anti-praja2 antibody and anti-β actin antibodies. (b) Cumulative analysis of praja2 levels in each category of tissue lysates. *P<0.01 versus astrocytoma II, Student’st-test. (c) Expression analysis of praja2 mRNA by RT–qPCR. The graph shows the enhancement of praja2 transcript levels in astrocytoma II and GBM lesions. Levels of praja2 mRNA in normal human brain served as baseline. *Statistically significant values at REST 2009 analysis, Student’st-test. (d) Tissue sections from human astrocytoma II and GBM were stained with hematoxylin/eosin (H & E) or immunostained with anti-praja2 and anti-MOB1 antibody, and analysed by light microscopy. Scale bar, 25 μm. (e) GBM and astrocytoma tissue sections were immunostained with anti-YAP and anti-phospho YAP antibody. Enlarged sections are shown on the right of each pair of images. Scale bar, 25 μm. Figure 6: praja2 is overexpressed in high-grade human glioma. ( a ) Lysates from tissue samples of astrocytoma (grade II) and GBM were immunoblotted with anti-praja2 antibody and anti-β actin antibodies. ( b ) Cumulative analysis of praja2 levels in each category of tissue lysates. * P <0.01 versus astrocytoma II, Student’s t -test. ( c ) Expression analysis of praja2 mRNA by RT–qPCR. The graph shows the enhancement of praja2 transcript levels in astrocytoma II and GBM lesions. Levels of praja2 mRNA in normal human brain served as baseline. *Statistically significant values at REST 2009 analysis, Student’s t -test. ( d ) Tissue sections from human astrocytoma II and GBM were stained with hematoxylin/eosin (H & E) or immunostained with anti-praja2 and anti-MOB1 antibody, and analysed by light microscopy. Scale bar, 25 μm. ( e ) GBM and astrocytoma tissue sections were immunostained with anti-YAP and anti-phospho YAP antibody. Enlarged sections are shown on the right of each pair of images. Scale bar, 25 μm. Full size image We then asked whether enhanced expression of praja2 in glioma tissues was associated with changes in the intracellular distribution of the ligase. Immunofluorescence analysis of glioma tissues is shown in Supplementary Fig. S8 . In astrocytoma tissue, moderate praja2 staining was homogeneously distributed at the cell periphery ( Supplementary Fig. S8a,b ). As expected, strong praja2 staining was observed in GBM cells ( Supplementary Fig. S8a,b ). This staining was diffusely distributed throughout the cytoplasm, with some concentration at the perinuclear membrane and the nuclear compartment. Conversely, the MOB1 immunofluorescent signal was intense in astrocytoma cells, whereas only a slight signal was detected in GBM lesions ( Supplementary Fig. S8c,d ). Note that GBM sections contain heterogenous cell populations marked by quite different levels of praja2 and MOB1, possibly reflecting the high rate of genomic instability that defines these tumours. Increased levels of praja2 in GBM lesions were linked to significantly decreased YAP phosphorylation ( Fig. 6e ). The unmodified YAP accumulated in the nuclear compartment ( Fig. 6e ). In contrast, astrocytoma tissues present high levels of phosphorylated YAP, which is mostly distributed throughout the cytoplasm ( Fig. 6e ). Here, we report a mechanism of signal attenuation in human GBM based on proteolytic turnover of components of an oncosuppressive pathway. We find that praja2 directly binds to and ubiquitylates MOB1, the regulatory component of the LATS1/2 kinases of the Hippo pathway. Degradation of ubiquitylated MOB1 by the proteasome inhibits this signalling cascade, favoring GBM growth. Proteolysis of cellular proteins by the UPS is a sophisticated mechanism controlling complex biological interactions that underlie cell survival, growth and metabolism. Accordingly, disregulation of the UPS is causally implicated in a wide variety of human diseases, including neurodegeneration and cancer. Modulating overall UPS activity is a therapeutic strategy currently being tested for treatment of several human disorders [41] . However, non-specific side effects and toxicity problems limit its use. An alternative approach, targeting the levels or activity of specific E3 ligases, is an attractive and, perhaps, more effective therapeutic strategy [42] . The E3-ubiquitin ligase MDM2 represents the prototype target of inhibitors that selectively interfere with the ubiquitylation processes in human tumours. MDM2 is a transcriptional target of p53 and tightly regulates p53 levels by marking p53 for UPS degradation [43] . This constitutes a negative feed-back loop that controls the p53-dependent stress response. Decreased levels of p53 are found in many human cancers, resulting from genetic inactivation, viral infection or amplification of the MDM2 gene [44] . Preventing MDM2–p53 interaction with small-molecule drugs restores normal p53 activity. This therapy is currently being tested in haematological and solid malignancies [45] . Changes in the expression profile of components of the ubiquitin ligase complexes have been reported in diverse tumours [20] . UbcH10, an ub-conjugating enzyme that regulates cell cycle progression, is upregulated in high-grade astrocytoma [46] . Conversely, the tumour suppressor F-box protein Fbxw7, a component of the Skp1-Cul1-F-box E3-ubiquitin ligase complex, is downregulated in high-grade glioma, and serves as prognostic biomarker for survival in glioma patients [47] . Somatic mutations of ubiquitin ligases have been identified in GBM and in other human malignancies, further supporting a pathogenic role of deregulated UPS system in brain tumours [48] , [49] . Our findings identify praja2 as a novel cancer-associated gene whose expression is upregulated in high-grade glioma. The expression profile of praja2 in tissue biopsies of astrocytoma and GBM lesions is consistent with a direct correlation between the levels of the ligase and the malignant phenotype of the tumour. At the mechanistic level, we identified MOB1, the regulatory component of the LATS1/2 kinases, as a critical praja2 substrate. MOB1 family members (MOB1A and MOB1B) are products of highly conserved genes originally identified as regulators of mitotic exit and cytokinesis in yeast, and later reported as tumour suppressors and components of the Hippo-NDR/LATS pathway [25] . MOB1 interacts with and activates LATS1/2 kinases. The MOB1/LATS kinase complex phosphorylates and inactivates YAP, a transcription factor that controls entry into the cell cycle of quiescent cells. Phosphorylated YAP is recruited and ubiquitylated by the SCF (beta-TRCP) E3-ubiquitin ligase complex. Ubiquitylated YAP is degraded through the proteasome [50] . The Hippo pathway can also be attenuated by proteolytic turnover of the LATS1 Kinase. LATS1 is ubiquinitated by the HECT class E3-ubiquitin ligase ITCH, which interacts with the PPxY motifs of LATS1 through its WW domains. Proteolysis of ubiquitylated LATS1 enhances cell growth, induces epithelial-mesenchymal transition and increases tumorigenicity [51] , [52] . In the work described above, we report that the regulatory component of the LATS1 kinase, MOB1, is degraded by praja2 through the UPS. Proteolysis of MOB1 by praja2 attenuates the Hippo cascade and enhances proliferation of glioblastoma cells. As MOB1 interacts with NDR1/2 kinases, this suggests that praja2 may also impact on the NDR1/2-dependent signalling cascade [32] . This mechanism operates in vivo ; downregulation of MOB1 restored the proliferative activity of praja2-silenced GBM cells and sustained tumour growth. By removing the inhibitory constraint imposed by Hippo, praja2 would favour YAP-dependent gene transcription, coupling the UPS pathway to GBM growth ( Fig. 7 ). Notably, we found that MOB1 levels inversely correlate with praja2 abundance and glioma malignancy, supporting the role of praja2 in control of MOB1 stability in vivo . Moreover, upregulation of praja2 in GBM lesions is linked to significant inhibition of the Hippo pathway, confirming the mechanistic link between praja2, Hippo pathway and GBM in vivo . 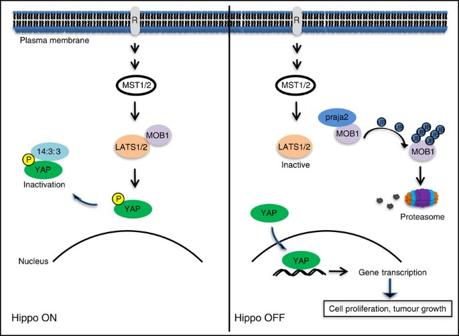Figure 7: Schematic diagram of the role of praja2 in the Hippo pathway. praja2-directed ubiquitylation of MOB1 and its consequent degradation by the proteasome attenuates LATS1/2 kinase activity, preventing phosphorylation and inactivation of YAP. Unphosphorylated YAP accumulates in the nucleus and drives gene transcription, promoting cell proliferation and tumour growth. Figure 7: Schematic diagram of the role of praja2 in the Hippo pathway. praja2-directed ubiquitylation of MOB1 and its consequent degradation by the proteasome attenuates LATS1/2 kinase activity, preventing phosphorylation and inactivation of YAP. Unphosphorylated YAP accumulates in the nucleus and drives gene transcription, promoting cell proliferation and tumour growth. Full size image Our results, taken together, identify the E3 ligase praja2 as a novel cancer-associated gene whose expression predicts the aggressive potential of glioma. Negative regulation of the Hippo pathway by praja2 constitutes a UPS-driven signalling circuit that sustains growth of glial cells carrying various oncogenic mutations. Unveiling the mechanism(s) regulating praja2 expression and activity in glioma cells and identifying additional relevant praja2 targets will contribute to our understanding of the role of UPS pathway in the development and progression of human GBMs. We expect this to inform the design of more effective target-oriented therapeutic strategies for aggressive human GBM. Cells and tissues The human embryonic kidney cell line (HEK293) was cultured in DMEM containing 10% fetal bovine serum (FBS) in an atmosphere of 5% CO 2 . The glioblastoma cell line U87MG (grade-IV) was purchased from the American Type Culture Collection and maintained in modified Eagle’s medium supplemented with 10% heat inactivated fetal calf serum and 2 mM L -glutamine, 100 IU ml −1 penicillin, 100 μgml −1 streptomycin, 1x non-essential amino-acid, 1 mM sodium pyruvate, at 37 °C, 5% CO 2 and 95% of humidity. Primary glioblastoma cell lines (FNP8 and NMDP7) were prepared from enzymatic digestion of bioptic samples surgically removed from Neuromed patients. All patients gave their informed consents and were shown to carry glioblastoma multiforme (according to WHO classsification). All tumours were positive for vimentin, GFAP (glial fibrillary acidic protein) and EGFR. Transfection of plasmids and siRNAs Vectors encoding for wild-type or mutant praja2, ubiquitin, MOB1A and MOB1B were described previously [53] , [54] . Transfection efficiency was monitored by including a GFP vector in the trasfection mixture. SMARTpool siRNAs targeting distinct segments of coding regions of praja2 and MOB1 were purchased from Dharmacon. The following are the siRNA sequences (Thermo Scientific) targeting human praja2: sequence 1: 5′-GAAGCACCCUAAACCUUGA-3′; sequence 2: 5′-AGACUGCUCUGGCCCAUUU-3′; sequence 3: 5′-GCAGGAGGGUAUCAGACAA-3′; sequence 4: 5′-GUUAGAUUCUGUACCAUUA-3′. The following are the siRNA sequences (Thermo Scientific) targeting human MOB1: sequence 1: 5′-AUGAAUGGGUUGCAGUUAA-3′; sequence 2: 5′-GCAGAUGGAACGAACAUAA-3′; sequence 3: 5′-GCACCAAAGUAUAUUGAUU-3′; sequence 4: 5′-GGUUAAAUGUUGAUACGAA-3′. siRNAs were transiently transfected using Lipofectamine 2000 (Invitrogen) at a final concentration of 100 pmol ml −1 of culture medium. For siRNA experiments, similar data were obtained using a mixture or four or two independent siRNAs. Antibodies and chemicals Goat and rabbit polyclonal antibodies directed against MOB1 were purchased from SantaCruz and Cell Signalling, and used at working dilutions of 1:300 (for immunostaining) and 1:1000 (for immunoblot); extracellular signal-regulated kinase 2 (ERK2) (dilution 1:3000), GST (dilution 1:5000),YAP (dilution 1:1000 for immunoblot and 1:300 for immunostaining), cyclin D1 (dilution 1:1000), cyclin B1 (dilution 1:1000) and cyclin E (dilution 1:1000) were purchased from SantaCruz; haemagglutinin epitope (HA.11, dilution 1:1000) was purchased from Covance; α-tubulin, γ-tubulin, flag and myc epitope (dilutions 1:3000) were purchased from Sigma; phospho(Ser127)YAP (dilution 1:1000), phospho(Ser909)LATS1 (dilution 1:1.000) and LATS1 (dilution 1:1000) were purchased from Cell Signalling; praja2 (dilution 1:5.000 for immunoblot and 1:300 for immunostaining) was purchased from Bethyl laboratories; polyclonal antibody directed against human praja2 (immunoblotting dilution 1:500; immunostaining dilution 1:300) was generated in rabbit using the following epitope: residues 60–250. Immunoprecipitation and pulldown assay Cells were homogenized and subjected to immunoprecipitation and immunoblot analyses as described previously [24] . GST fusions were expressed and purified from BL21 (DE3) pLysS cells. GST or GST–praja2, beads (20 μl) were incubated with 2 mg of cell lysate or with in vitro -translated [ 35 S]-labelled MOB1A in 200 μl lysis buffer (150 mM NaCl, 50 mM Tris-HCl at pH 7.5, 1 mM EDTA and 0.5% Triton X-100) in rotation at 4 °C overnight. Pellets were washed four times in lysis buffer supplemented with NaCl (0.4 M final concentration) and eluted in Laemmli buffer. Eluted samples were immunoblotted with the indicated antibody. In the case of GST/GST-MOB1A pulldowns, we precipitated praja2-flag expressed in HEK293 cells for 3 h (lysis buffer: 10 mM sodium phosphate pH 7.2, 150 mM NaCl, 0.5% Triton X-100 supplemented with standard protease inhibitors). Resin-associated complexes were washed at least four times with the lysis buffer and eluted with Laemmli sample buffer. In vitro ubiquitylation assay [ 35 S]-labelled MOB1A was synthesized in vitro using a TnT Quick coupled transcription/translation system (Promega) in the presence of 45 μCi of [ 35 S]-labelled methionine using as template a pcDNA3 vector carrying Myc/His-MOB1A transgene. The ubiquitylation assay was carried out as described previously [53] . Animals and tumour cell implantation Male CD1 nude mice (20–22 g body weight; Charles River, Calco, CO, Italy) were kept under controlled conditions (temperature, 22 °C; humidity, 40%) on a 12-h light/dark cycle with food and water ad libitum . Experiments were performed following the guidelines for animal care and use proposed by the National Institutes of Health (Bethesda, MD). Mice were subcutaneously implanted with 1 × 10 6 U87MG cells per 0.5 ml, under anaesthesia. The weight of subcutaneous tumours was assessed after 1 month. In another set of experiments, U87MG cells were stereotaxically implanted into the left caudate nucleus (by using the following coordinates: 0.6 mm anterior to the bregma; 1.7 mm lateral to the midline; and 4.5 mm ventral from the surface of skull of mice under ketamine (100 mg kg −1 , i.p. )/xylazine (10 mg kg −1 , i.p.) anaesthesia. Cells (0.3 × 10 6 cells per 5 μl) were implanted at an infusion rate of 1 μl min −1 . Immunohistochemistry Formalin-fixed, paraffin-embedded tissues from the tumours were selected. Representative slides of each tumour were stained with hematoxylin and eosin. Immunohistochemistry for praja2 and Ki67 (Ventana, Tucson, Ariz.) was performed automatically with a Nexes instrument (Ventana). Antibody detection was performed using a multilink streptavidin–biotin complex method, and antibodies were visualized by a diaminobenzidine chromagen method. Negative control samples were incubated with primary antibodies only. The number of Ki67-positive cells was determined in four random fields (1 cm 2 each) by using the ImageJ 1.31v software (National Institutes of Health). Stereological techniques for electron microscopic morphometry were applied to normal brain and brain tumour slides. Our aim was to obtain objective baseline data for the study of expression of praja2 in these tissues. The results, expressed mainly in numerical densities of positive cells in the control and pathological tissue revealed increasing gradients throughout grading of the tumour tissues. Each section was subjected to count stereology of cells positive for praja2. The counting was performed using a microscope (Axio Imager M1 microscope) equipped with software Image Pro Plus 6.2. This automatically calculates the density of praja2 positive cells per area (mm 2 ). To evaluate the expression of MOB1, YAP and phospho YAP in tumour cells, 4-m serial sections from representative blocks were cut, mounted on poly- L -lysine coated glass slides and used for the immunohistochemical staining. Representative sections were incubated with the anti-MOB1, anti-YAP and anti-phospho YAP antibodies. Subsequently, the slides were incubated with biotinylated secondary antibodies, peroxidase-labelled streptavidin (DAKO LSAB kit HRP, Carpinteria, CA) and chromogenic substrate diaminobenzidine (DAB, Vector Laboratories, Burlingame, USA) for the development of the peroxidase activity. Slides were counterstained with hematoxylin, dehydrated and cover-slipped with a synthetic mounting medium (Entellan, Merck, Germany). Only cells with a definite cytoplasmic staining were judged as positive for the MOB1 antibody, whereas for YAP and phospho-YAP nuclear and cytoplasmic positivity were evaluated, respectively. Small animal PET Imaging and data analysis Before PET studies, mice were injected in the tail vein with 9.5 MBq of 18 F-FLT, and were kept awake in a ventilated cage (26 °C) during a tracer uptake period of 60 min. Anaesthesia was performed with intraperitoneal administration of ketamine (100 mg kg −1 ) and xylazine (10 mg kg −1 ) (injection volume, 100 μl per 10 g) during the entire scanning period. Imaging was performed with the dedicated small animal PET scanner eXplore Vista GE Healthcare. The static PET data were acquired for 30 min. Image data sets were corrected for random coincidences, scatter and physical decay to the time of injection. No attenuation correction was applied. The measured reconstructed spatial resolution of the Explore Vista scanner is ~1.6 mm full-width at half maximum (FWHM) at the center of the field of view. The counting rates in the reconstructed images were converted to activity concentrations (SUV units) by use of a system calibration factor (1,035 Bq ml −1 per cps per voxel) derived from the imaging of a mouse-size water-equivalent phantom containing 18 F. Maximum (SUVmax) and mean (SUVmean) standardized uptake values (SUVs) (SUV=tissue activity (MBq per cc)/(injected dose (MBq)/body weight (g))), and the ‘metabolic volume’ of the lesions were calculated from the PET studies. Quantitative data were obtained using GE eXplore Vista software, on the base of a ‘region growing’ procedure, by adding all spatially connected voxels with SUV >50%. FLT uptake between control and siRNA-treated mice were compared. Immunofluorescence and confocal analysis Sections from human glioblastoma biopsies were subjected to double staining with DAPI and primary antibodies. Fluorescent signals were visualized using a Zeiss LSM 510 Meta argon/krypton laser scanning confocal microscope. Four images from each optical section were averaged to improve the signal-to-noise ratio. Images from a minimum of four sections per tumour and four different samples of each category of tumours were collected and analysed. Immunofluorescence on cultured cells was performed as described previously [24] . Fluorescence-activated cell sorting For cell cycle analysis, samples were labelled with propidium iodide. Cells were fixed with 70% ethanol in phosphate-buffered saline (PBS) and routinely kept at +4 C° overnight. Cells were washed twice with PBS, resuspended in PBS containing 40 μg ml −1 propidium iodide (Sigma), 7 units μl −1 RNase DNase-free (Eppendorf) and incubated at room temperature for 20 min. Cells were analysed using a CyAn ADP flow cytometer (Dako Cytomation, Ely, UK) using Summit software. Results are presented as mean±s.e.m. of three separate experiments. In vitro protein binding assays GST hybrid proteins were expressed in Escherichia coli (strain BL21). Induction, cell lysis and affinity purification of hybrid proteins were performed as recommended by the supplier of the pGEX vectors (GE Healthcare). GST hybrid proteins (GST, GST-MOB1A) immobilized on glutathione beads were incubated for 3 h with cell lysates from HEK293 cells transiently expressing flag-praja2. Resin-associated complexes were washed at least four times with the standard lysis buffer (10 mM sodium phosphate pH 7.2, 150 mM NaCl, 0.5% Triton X-100) and eluted with Laemmli sample buffer (2% SDS, 50 mM Tris-HCl pH 6.8, 0.2 mg ml −1 bromphenol blue, 0.1 M DTT, 10% (v/v) glycerol). How to cite this article: Lignitto, L. et al. Proteolysis of MOB1 by the ubiquitin ligase praja2 attenuates Hippo signalling and supports glioblastoma growth. Nat. Commun. 4:1822 doi:10.1038/ncomms2791 (2013).